Highly efficient non-rare-earth red emitting phosphor for warm white light-emitting diodes Mn 4+ -activated fluoride compounds, as an alternative to commercial (oxy)nitride phosphors, are emerging as a new class of non-rare-earth red phosphors for high-efficacy warm white LEDs. Currently, it remains a challenge to synthesize these phosphors with high photoluminescence quantum yields through a convenient chemical route. Herein we propose a general but convenient strategy based on efficient cation exchange reaction, which had been originally regarded only effective in synthesizing nano-sized materials before, for the synthesis of Mn 4+ -activated fluoride microcrystals such as K 2 TiF 6 , K 2 SiF 6 , NaGdF 4 and NaYF 4 . Particularly we achieve a photoluminescence quantum yield as high as 98% for K 2 TiF 6 :Mn 4+ . By employing it as red phosphor, we fabricate a high-performance white LED with low correlated colour temperature (3,556 K), high-colour-rendering index ( R a =81) and luminous efficacy of 116 lm W −1 . These findings show great promise of K 2 TiF 6 :Mn 4+ as a commercial red phosphor in warm white LEDs, and open up new avenues for the exploration of novel non-rare-earth red emitting phosphors. Solid-state white light-emitting diodes (LEDs) are next-generation lighting devices for replacing the traditional incandescent and fluorescent lamps due to their superior properties such as energy-saving, robust, long-lifetime and environment-friendly features [1] , [2] , [3] , [4] , [5] , [6] , [7] , [8] , [9] , [10] , [11] , [12] , [13] . Nowadays, a blue diode chip combined with Y 3 Al 5 O 12 :Ce 3+ (YAG:Ce 3+ ) yellow phosphor is still the most mature method for fabricating commercial white LEDs. YAG:Ce 3+ is an excellent phosphor for blue-chip excitation with high photoluminescence (PL) quantum yield (QY) and good thermal stability. However, because of the lack of red light component in the emission of YAG:Ce 3+ , it is notoriously difficult to make warm white LEDs with high-colour-rendering index (CRI, R a >80) and low correlated colour temperature (CCT<4,500 K), both of which are key requirements for some important applications such as indoor lighting. This difficulty can be completely overcome by adding a suitable red phosphor in LEDs to complement the red light component. To this end, great efforts have been made to exploit novel rare-earth-doped red phosphors, and the most successful materials are Eu 2+ - or Ce 3+ -doped (oxy)nitride compounds [14] , [15] , [16] , [17] , [18] , [19] , typically CaAlSiN 3 :Eu 2+ (ref. 20 ). Albeit commercialized in recent years, the CaAlSiN 3 :Eu 2+ phosphor still has several drawbacks: First, its emission spectrum is very broad (full-width at half-maximum=~80 nm) and a large part of the spectrum is beyond 650 nm in wavelength and insensitive to human eyes [20] , [21] , [22] , thereby decreasing the luminous efficiency of radiation (LER) [23] . Second, the absorption of the phosphor covers the spectral range of ~200–650 nm; therefore serious re-absorption will take place when this phosphor is mixed with other green or yellow phosphors, which causes colour change and lower luminous efficacy of LEDs [24] , [25] . Third, the rigorous synthesis conditions of nitride compounds increase its production cost. Generally, CaAlSiN 3 :Eu 2+ phosphor was prepared by firing a powder mixture of Si 3 N 4 , AlN, Ca 3 N 2 and EuN raw materials at 1,600–1,800 °C for 2 h under 0.5 MPa nitrogen atmosphere [26] . To circumvent the above drawbacks, an ideal red phosphor with relatively narrow absorption and emission bands, a high PL QY and low-production cost are highly desired for warm white LEDs. Mn 4+ belongs to transition metal ion with outer 3d 3 electron configuration. An interesting spectral feature of Mn 4+ is that it exhibits both broadband excitation and sharp emission lines due to its distinct electronic structure. Additionally, their optical properties are strongly influenced by local crystal field environments. For example, the excitation and emission peaks of Mn 4+ in oxide hosts are usually at ~300 and ~650 nm, respectively [27] , [28] , [29] . However, when Mn 4+ ions are situated at fluoride hosts with octahedral coordination, they exhibit the most intense broadband excitation at ~460 nm with a bandwidth of ~50 nm and very sharp emission lines peaking at ~630 nm as a result of weaker crystal field for Mn 4+ (refs 30 , 31 , 32 ). These unique optical characteristics meet the spectral requirements for an ideal red phosphor and thus enable the family of Mn 4+ -doped fluoride compounds as promising candidates of red emitting phosphors for blue-chip excited warm white LEDs with high LER. So far, most of previous efforts were devoted to the preparation and optical properties investigation of Mn 4+ -doped fluoride phosphors [30] , [31] , [32] , [33] , [34] , [35] . To the best of our knowledge, warm white LEDs based on Mn 4+ -doped red phosphors with a luminous efficacy higher than 90 lm W −1 , a prerequisite for further commercialization, had never been achieved before. The K 2 TiF 6 crystal has a hexagonal structure with P m1 space group, and the Ti 4+ ion is coordinated with six F − ions to form a regular octahedron [36] . It is a suitable host for Mn 4+ doping in view of the same valence and similar ionic radius between Ti 4+ (0.0605, nm with six coordination) and Mn 4+ (0.0530, nm with six coordination) [37] . Currently, it remains a great challenge to synthesize this phosphor with high PL QY through a convenient chemical route. Particularly, the synthetic approaches previously established are not practical for its low-cost mass production. For instance, K 2 TiF 6 :Mn 4+ was usually prepared via cocrystallization [30] , [35] , [38] , [39] . The fluoride host and source materials of Mn 4+ (generally alkali metal hexafluoromanganates) were dissolved in concentrated hydrofluoric acid (HF) solution and then evaporated slowly to dryness. As such, the whole preparation process was time-consuming, and massive evaporated HF gas must be handled with great care. Another approach for the synthesis of this phosphor is to etch TiO 2 in HF solution mixed with KMnO 4 (ref. 34 ). However, its production yield is very low because metal oxides usually have large solubility in concentrated HF solution. Therefore, a general but convenient synthesis method is highly demanded for K 2 TiF 6 :Mn 4+ as well as other Mn 4+ -activated fluoride red phosphors. On the other hand, a comprehensive understanding of the electronic structure and optical properties of Mn 4+ emitters in fluoride phosphors, which is crucial to improving their PL QYs for further applications, is still lacking. For instance, the mechanism behind the abnormal temperature-dependent PL intensity behaviour of Mn 4+ ions remains unclear till now [27] . An in-depth investigation of the optical properties and device performance of Mn 4+ -activated phosphors will promote the application of this cheap and abundant resource in the field of solid-state lighting, thus reduce the consumption of expensive rare-earth such as Eu. In this work, we propose a unique method based on cation exchange reaction for preparing highly efficient K 2 TiF 6 :Mn 4+ red phosphor with a PL QY up to 98%. We also demonstrate that such an approach is general to the synthesis of various Mn 4+ -activated fluoride phosphors such as K 2 SiF 6 :Mn 4+ , NaGdF 4 :Mn 4+ and NaYF 4 :Mn 4+ . Particularly, the fine electronic/vibronic structures and excited-state dynamics of Mn 4+ ions in K 2 TiF 6 host are revealed for the first time by means of high-resolution optical spectroscopy. By employing K 2 TiF 6 :Mn 4+ as red phosphor, we realize a high-performance warm white LED with low CCT (3,556 K), high CRI ( R a =81) and luminous efficacy of 116 lm W −1 , which presents a substantial advance towards its commercial application. Synthesis strategy The main difficulty for synthesizing Mn 4+ -activated fluoride compounds lies in that Mn has diverse valence states, thus valence change of Mn 4+ often occurs during synthesis, resulting in undesired byproducts. Although the doping of Mn 4+ has been realized in oxide compounds through solid-state reaction at high temperature, it is unpractical for synthesizing Mn 4+ -activated fluoride compounds through this route because hazard and corrosive HF gas was used to prevent the oxidation of products [40] . In contrast, cation exchange reaction has been proved to be a convenient method for lanthanide doping in nano-sized fluoride crystals [41] , [42] . It was well established that efficient cation exchange can only take place in nano-sized materials [43] , [44] . Interestingly, we recently found that the cation exchange approach can also be applicable for the synthesis of micrometre-sized materials with unusually fast reaction rate. To demonstrate this, we employed this approach to the synthesis of K 2 TiF 6 :Mn 4+ microcrystals. The preparation was carried out by simply mixing K 2 TiF 6 host with a small volume of HF solution dissolved with K 2 MnF 6 powders. After stirring for 20 min, a muddy mixture was formed, and then heated at 70 °C for 3 h, which afforded the final product of K 2 TiF 6 :Mn 4+ . It is worthy of emphasizing that only a small portion of K 2 TiF 6 raw powders was dissolved in HF solution containing Mn 4+ ions (the solubility of K 2 TiF 6 in 49 wt.% HF solution is ~0.17 g ml −1 at room temperature (RT)), and cocrystallization of K 2 TiF 6 :Mn 4+ may occur for this portion once the mixture was directly heated to dryness. However, for the undissolved portion, we assume that the cation exchange reaction, namely, the replacement of Ti 4+ ions in K 2 TiF 6 crystals with the Mn 4+ ions in the solution, is responsible for the doping of Mn 4+ . To verify our hypothesis, we carried out a proof-of-concept experiment. The K 2 TiF 6 powders were immersed in HF solution containing Mn 4+ ions (the atom percent of Mn is 5.50%). After cation exchange reaction at RT for 3 min under stirring, the powders were isolated instantly through vacuum filtration. It was observed that the colour of the mixture solution changed from brown to light-yellow, indicating a remarkable decrease of the Mn 4+ concentration in the solution. Accordingly, the colour of the powders was observed to change from white to yellow after cation exchange ( Fig. 1a,b ). This reaction process was dynamically demonstrated by illuminating the K 2 TiF 6 powders with 455-nm blue light under stirring, which showed a remarkable increase in red light emission within 3 min ( Supplementary Movie 1 ). The X-ray diffraction (XRD) pattern of the final powder product confirmed that it remained pure in hexagonal K 2 TiF 6 phase ( Supplementary Fig. 1 ). Under illumination with the 455-nm light, the powders show bright red emission, indicating the successful doping of Mn 4+ into the crystal lattice of K 2 TiF 6 . The Mn 4+ concentration in the as-synthesized powders was determined to be 3.70 at.% (that is, 67% of the Mn 4+ ions in the precursor solution) by means of inductively coupled plasma–atomic emission spectroscopy (ICP–AES). The observation of such a high Mn 4+ content within the short reaction time shows unambiguously that the cation exchange occurred with an unusually fast reaction rate. 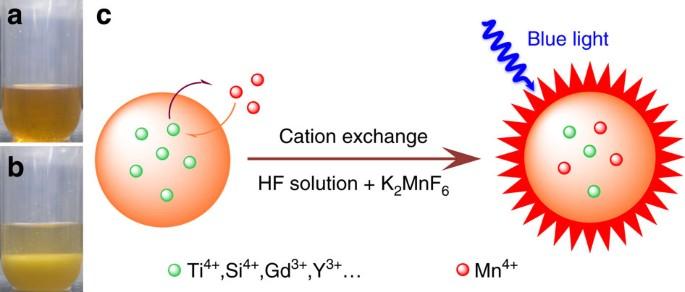Figure 1: Synthesis of Mn4+-activated red phosphors based on the strategy of cation exchange. Photographs of the HF solution dissolved with K2MnF6crystals (a) and the same solution containing K2TiF6powders after cation exchange reaction for 3 min (b). (c) Schematic illustration of the cation exchange procedure for synthesizing Mn4+-activated fluoride compounds. Figure 1c schematically illustrates this cation exchange procedure for synthesizing Mn 4+ -activated fluoride compounds. Figure 1: Synthesis of Mn 4+ -activated red phosphors based on the strategy of cation exchange. Photographs of the HF solution dissolved with K 2 MnF 6 crystals ( a ) and the same solution containing K 2 TiF 6 powders after cation exchange reaction for 3 min ( b ). ( c ) Schematic illustration of the cation exchange procedure for synthesizing Mn 4+ -activated fluoride compounds. Full size image Different from the traditional cocrystallization method, our strategy based on cation exchange shows two distinct advantages: (1) The consumption of HF solution per gram of K 2 TiF 6 :Mn 4+ product (~0.36 ml g −1 ) is 17 times lower than that of cocrystallization method (~6 ml g −1 ), which is very beneficial to the waste processing of the hazard HF gas produced during synthesis; (2) The synthetic time is significantly shortened and the whole procedure is well controlled, which are crucial for mass production of K 2 TiF 6 :Mn 4+ . This strategy can be further extended for synthesizing other Mn 4+ -activated fluoride materials such as K 2 SiF 6 :Mn 4+ , NaGdF 4 :Mn 4+ and NaYF 4 :Mn 4+ . Similarly, XRD patterns and PL spectra of these samples show the pure crystalline phase of each host and typical sharp emissions of Mn 4+ at ~630 nm on 455-nm excitation ( Supplementary Figs 2–4 and Methods ). All these results prove that the proposed cation exchange strategy is universal for the synthesis of Mn 4+ -activated fluoride phosphors. Structural characterization We synthesized five K 2 TiF 6 :Mn 4+ samples with various Mn 4+ concentrations through cation exchange route. Compositional analyses through ICP–AES reveal that the Mn 4+ concentrations of the samples were 0.72, 1.40, 2.10, 5.50 and 6.50 at.%, respectively. The XRD patterns of these five samples along with the pure K 2 TiF 6 sample and K 2 MnF 6 crystal are compared in Fig. 2a . All the diffraction peaks of K 2 TiF 6 :Mn 4+ samples can be indexed to P m1 space group of hexagonal K 2 TiF 6 phase (JCPDS No. 00-008-0488). No traces of K 2 MnF 6 residual and other impurity phases were observed. The crystal structure of K 2 TiF 6 viewed from [110] direction is shown in Fig. 2b . Each Ti 4+ ion is surrounded by six F − ions resulting in only one kind of TiF 6 2− octahedral structure. Notably, the K + ion is at the centre of 12 nearest neighbour F − ions forming a nearly regular polyhedron. The scanning electron microscope image of the 5.50 at.% sample indicates that the particle size is primarily in the range of 10–20 μm ( Fig. 2c ). The sample shows a uniform yellow tint under natural light illumination ( Fig. 2d ). While under blue light (455 nm) excitation, it emits brilliant red light, indicating high emission efficiency ( Fig. 2e ). 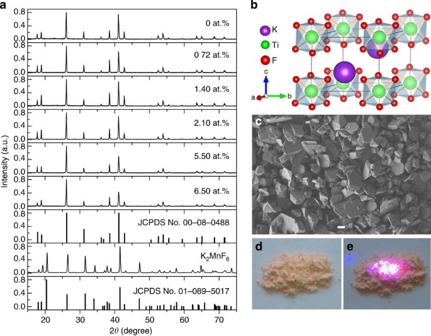Figure 2: Structure and morphology of the synthesized K2TiF6:Mn4+phosphors. (a) X-ray diffraction patterns of the K2MnF6crystal and K2TiF6samples doped with various Mn4+contents. All diffraction peaks match well with the standard patterns of K2MnF6(JCPDS No. 01-089-5017) and tetragonal-phase K2TiF6(JCPDS No. 00-008-0488), respectively. (b) Crystal structure of K2TiF6unit cell viewed in [110] direction. (c) Representative scanning electron microscope image of the K2TiF6:Mn4+(5.5 at.%) sample. Scale bar, 10 μm. Photographs of the K2TiF6:Mn4+(5.50 at.%) sample under natural light (d) and 455-nm blue light (e) illumination, respectively. a.u., arbitrary unit. Figure 2: Structure and morphology of the synthesized K 2 TiF 6 :Mn 4+ phosphors. ( a ) X-ray diffraction patterns of the K 2 MnF 6 crystal and K 2 TiF 6 samples doped with various Mn 4+ contents. All diffraction peaks match well with the standard patterns of K 2 MnF 6 (JCPDS No. 01-089-5017) and tetragonal-phase K 2 TiF 6 (JCPDS No. 00-008-0488), respectively. ( b ) Crystal structure of K 2 TiF 6 unit cell viewed in [110] direction. ( c ) Representative scanning electron microscope image of the K 2 TiF 6 :Mn 4+ (5.5 at.%) sample. Scale bar, 10 μm. Photographs of the K 2 TiF 6 :Mn 4+ (5.50 at.%) sample under natural light ( d ) and 455-nm blue light ( e ) illumination, respectively. a.u., arbitrary unit. Full size image To reveal whether the Mn 4+ ions are located on the surface of or distributed uniformly across the K 2 TiF 6 :Mn 4+ crystals synthesized through cation exchange, we first compared the XRD patterns of the samples and found a slight shift of the diffraction peaks to higher angles with the increase of Mn 4+ doping concentrations ( Fig. 2a and enlarged XRD patterns in Supplementary Fig. 5a ). Accordingly, the fitted cell volume of the samples by the JADE software also decreases from 133.43 Å 3 for the pure sample to 133.04 Å 3 for the 6.50 at.% sample ( Supplementary Fig. 5b–d ). This observation is consistent with the expected structural change induced by the substitution of a smaller cation (Mn 4+ , 0.0530, nm) for a larger cation (Ti 4+ , 0.0605, nm) in the crystalline lattice. To investigate the Mn 4+ distribution in the crystals, we synthesized a 6.83 at.% K 2 TiF 6 :Mn 4+ sample through cation exchange for 20 min and washed this sample with HF solution (16 wt.%) to dissolve the surface of the crystals ( Supplementary Methods ). The colour of the crystals before and after washing is nearly the same ( Supplementary Fig. 6a–c ) and ICP–AES analyses show that the Mn 4+ concentration in the crystals remains nearly unchanged (6.96 at.%) after being washed twice. On the contrary, in a control experiment, the Mn 4+ concentration was found to decrease significantly from 0.45 to 0.02 at.% in the sample synthesized through cation exchange for only 10 s, which was also corroborated by the disappearance of red light emission for this sample after acid-washing treatment ( Supplementary Fig. 6d–f ). These results exclude the possibility of the Mn 4+ aggregation on the surface of the 6.96 at.% sample and suggest that Mn 4+ ions are distributed uniformly across the crystals. To further visualize the Mn 4+ distribution in the crystals, we carried out scanning transmission electron microscopy and energy dispersive spectroscopy analyses for the 6.96 at.% sample. Both elemental line scanning and mapping measurements show similar concentration distribution of the Mn to that of the Ti element ( Supplementary Fig. 7 ). The molar ratio of Mn to Ti was roughly estimated to be ~10% based on the calibrated signal intensities of energy dispersive spectroscopy, which is basically consistent with the Mn 4+ concentration (6.96 at.%) measured by ICP–AES. All above results prove that Mn 4+ ions are distributed uniformly across the crystals synthesized through cation exchange for 20 min. PL QY PL QY is a key parameter to evaluate a phosphor material. It is defined as the ratio of emitted photons to absorbed ones. For commercial phosphors such as YAG:Ce 3+ , the PL QY is usually larger than 90%. Unfortunately, currently no experimental PL QY is available for K 2 TiF 6 :Mn 4+ . We measured the absolute PL QY of the samples using an integrating sphere at RT and the results are listed in Table 1 . The samples doped with the Mn 4+ concentration of 5.50 at.% or lower show extremely high PL QYs ranging from 93 to 98%, which are comparable or superior to that of commercial YAG:Ce 3+ phosphor. As the Mn 4+ concentration increased from 5.50 to 6.50 at.%, the QY decreased dramatically from 93 to 78%, due to the concentration quenching effect at high doping concentration. We also measured RT PL decays from the emitting state 2 E g in these samples ( Supplementary Fig. 8 ), and each PL decay time was determined based on single exponential fit of the decay ( Table 1 ). It shows clearly that the PL lifetime of the 6.50 at.% sample is significantly shorter than those of other samples, indicating the largest non-radiative transition probability and thus the lowest PL QY of this sample. It is worthy of emphasizing that no decline of PL QYs was observed for these five samples after being kept at ambient conditions for over 1 year. This indicates that the K 2 TiF 6 :Mn 4+ phosphor is stable in the air. Table 1 Photoluminescence quantum yields (PL QYs) and lifetimes of the 2 E g state measured at room temperature for K 2 TiF 6 :Mn 4+ samples. Full size table Electronic and vibronic structures of Mn 4+ When Mn 4+ ions are situated at hosts with octahedral coordination, the dependence of energy levels of Mn 4+ on crystal field strength can be well illustrated by Tanabe-Sugano energy diagram ( Fig. 3a ) [45] . It shows clearly that the energies of most multiplets are strongly dependent on crystal field strength except 2 T 1 and 2 E g levels. Particularly, the optical characteristics of Mn 4+ in fluoride hosts can be inferred from their configurational coordinate diagrams ( Fig. 3b ) [46] . The 2 E g , 2 T 1 , 2 T 2 and 4 A 2 levels are derived from the electronic orbital, whereas the 4 T 1 and 4 T 2 levels are formed from another orbital [46] . As such, a large lateral displacement can be observed between the parabolas of ground state 4 A 2 and 4 T 1 (or 4 T 2 ), while a small displacement between the parabolas of 4 A 2 and 2 E g (or 2 T 1 , 2 T 2 ). Larger displacement implies stronger electron–phonon interaction (namely, larger Huang-Rhys factor) and thus larger spectral bandwidth of the transition [46] . Additionally, according to the spin selection rule of Δ S =0, the transitions between 4 T 1 , 4 T 2 and ground 4 A 2 levels are spin-allowed, thus intense excitation or absorption bands with relatively large bandwidths are expected between these levels. On excitation to 4 T 1 or 4 T 2 levels, the excited ions usually relax non-radiatively to 2 E g followed by the spin-forbidden 2 E g → 4 A 2 transition characterized by sharp emission lines. 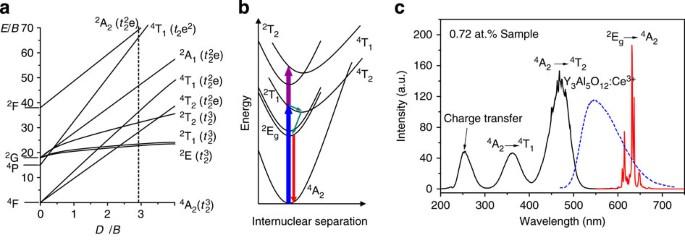Figure 3: Energy levels and optical spectra of Mn4+emitters in fluoride phosphors. (a) Tanabe-Sugano energy diagram of a 3d3system in an octahedral crystal field. (b) Configurational coordinate diagram for Mn4+ions in fluoride hosts. (c) Room temperature excitation and emission spectra of the K2TiF6:Mn4+(0.72 at.%) sample. The dashed line displays the emission spectrum of commercial Y3Al5O12:Ce3+yellow phosphor. a.u., arbitrary unit. Figure 3: Energy levels and optical spectra of Mn 4+ emitters in fluoride phosphors. ( a ) Tanabe-Sugano energy diagram of a 3d 3 system in an octahedral crystal field. ( b ) Configurational coordinate diagram for Mn 4+ ions in fluoride hosts. ( c ) Room temperature excitation and emission spectra of the K 2 TiF 6 :Mn 4+ (0.72 at.%) sample. The dashed line displays the emission spectrum of commercial Y 3 Al 5 O 12 :Ce 3+ yellow phosphor. a.u., arbitrary unit. Full size image We measured the RT excitation and emission spectra of K 2 TiF 6 :Mn 4+ and the results are in good agreement with the above predicted optical characteristics. There are three intense excitation bands of K 2 TiF 6 :Mn 4+ (0.72 at.%) in the range of 200–550 nm ( Fig. 3c ). The 362 and 468 nm bands are due to the spin-allowed 4 A 2 → 4 T 1 and 4 A 2 → 4 T 2 transitions, respectively. The full-width at half-maximum of the 468-nm band is ~50 nm, which is even broader than that of blue-chip emission (~20 nm). More importantly, as shown in Fig. 3c , the spectral overlap between excitation of K 2 TiF 6 :Mn 4+ and emission of YAG:Ce 3+ is negligibly small. Hence, serious re-absorption that often occurs between (oxy)nitride red phosphors and yellow (or green) phosphors in warm white LEDs can be avoided. The excitation band at 255 nm most likely originates from the charge transfer transition between F − and Mn 4+ ions [47] . The red emission originating from the spin-forbidden 2 E g → 4 A 2 transition is composed of several sharp lines distributed in the spectral range of 610–650 nm with the strongest peak at 631.5 nm ( Fig. 3c ). Such an emission pattern differs greatly from those of (oxy)nitride red phosphors that usually exhibit considerable emissions over 650 nm, and thus enables the fabrication of warm white LEDs with a higher LER. A clear depiction of the electronic and vibronic energy diagram of Mn 4+ in K 2 TiF 6 host is essential for understanding the optical behaviours and application of this phosphor. The optical transitions of Mn 4+ are sensitive to their local coordination, and the energy level splitting is determined by the local symmetry of the crystallographic site occupied by Mn 4+ ions. When Mn 4+ ions are doped into the crystal lattice of K 2 TiF 6 , they most probably substitute for Ti 4+ ions with local site symmetry of D 3d (ref. 36 ), descending from O h . Based on group theory [46] , we first analysed the effect of this symmetry descending on energy level splitting. Then the spin–orbit interaction was taken into account. Detailed energy levels of Mn 4+ at the site symmetry of D 3d were deduced and plotted in Fig. 4a . It can be seen that both 2 E g and 4 A 2 states split into two sublevels due to spin–orbit interaction, and emissions from lower and upper sublevels of 2 E g were denoted as zero-phonon lines (ZPLs) of R 1 and R 2 , respectively. 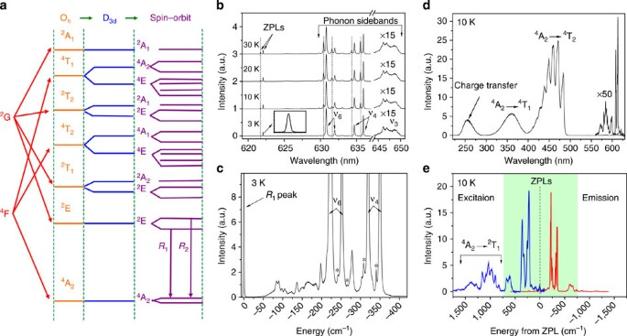Figure 4: High-resolution electronic and vibronic spectra of K2TiF6:Mn4+phosphor. (a) Deduced energy level splitting of Mn4+ions at a crystallographic site of D3dsymmetry. (b) High-resolution photoluminescence spectra of the K2TiF6:Mn4+(0.72 at.%) sample measured at 3–30 K on 460-nm excitation. The inset shows the enlarged R1peak of the zero-phonon lines (ZPLs) at 3 K. (c) Enlarged weak emission peaks at 3 K in the range of 0–400 cm−1shifting from the R1line (the energy of R1is set to zero). The peaks indicated by asterisks are the residual emissions coupled to the upper sublevel of2Eg. (d) Excitation spectrum of the K2TiF6:Mn4+(0.72 at.%) sample measured at 10 K when monitoring the dominant emission at 631 nm. (e) Comparison of the vibronic excitations of4A2→2T1,2Egat ~600 nm and the vibronic emissions of2Eg→4A2at 10 K (the energy of the R1line is set to zero). The vertical dashed lines inbandeare the guidance for the eye. a.u., arbitrary unit. Figure 4: High-resolution electronic and vibronic spectra of K 2 TiF 6 :Mn 4+ phosphor. ( a ) Deduced energy level splitting of Mn 4+ ions at a crystallographic site of D 3d symmetry. ( b ) High-resolution photoluminescence spectra of the K 2 TiF 6 :Mn 4+ (0.72 at.%) sample measured at 3–30 K on 460-nm excitation. The inset shows the enlarged R 1 peak of the zero-phonon lines (ZPLs) at 3 K. ( c ) Enlarged weak emission peaks at 3 K in the range of 0–400 cm −1 shifting from the R 1 line (the energy of R 1 is set to zero). The peaks indicated by asterisks are the residual emissions coupled to the upper sublevel of 2 E g . ( d ) Excitation spectrum of the K 2 TiF 6 :Mn 4+ (0.72 at.%) sample measured at 10 K when monitoring the dominant emission at 631 nm. ( e ) Comparison of the vibronic excitations of 4 A 2 → 2 T 1 , 2 E g at ~600 nm and the vibronic emissions of 2 E g → 4 A 2 at 10 K (the energy of the R 1 line is set to zero). The vertical dashed lines in b and e are the guidance for the eye. a.u., arbitrary unit. Full size image To further reveal the electronic and vibronic structure of Mn 4+ in K 2 TiF 6 crystal, we performed high-resolution PL measurement for the K 2 TiF 6 :Mn 4+ (0.72 at.%) sample at 3–30 K ( Fig. 4b ). The extremely low temperature can avoid thermal broadening of the spectral bands for more reliable assignment of energy levels. At 30 K, two weak and sharp emission peaks centred at 622.08 and 621.70 nm, which were also observed in the excitation spectrum, and can be unquestionably assigned to R 1 and R 2 ZPLs of the 2 E g → 4 A 2 transition, respectively. As theoretically predicted in Fig. 4a , four ZPLs are expected for the 2 E g → 4 A 2 transition due to double splitting of both 2 E g and 4 A 2 states. However, we cannot find such a pattern even in the enlarged region around the R 1 peak (inset of Fig. 4b ), due most possibly to the extremely small crystal field splitting of 4 A 2 that is beyond the spectral resolution of our spectrometer. For instance, the energy level splitting of 4 A 2 in Al 2 O 3 :Mn 4+ crystal was only ~0.39 cm −1 (ref. 28 ). With further decreasing the temperature, the intensity of the R 2 line (621.70 nm) decreased gradually and almost disappeared at 3 K due to the thermal de-population from the upper sublevel of 2 E g . The elimination of hot band emissions at 3 K enables more accurate identification of observed transitions. The weak intensity of the ZPLs of 2 E g → 4 A 2 is ascribed to their magnetic dipole nature. However, the coupling of electronic transition with vibronic modes may introduce odd-parity crystal field terms into the wavefunctions of 2 E g and thus render the vibronic transition allowed for electric dipole radiation. Therefore, phonon-coupled vibronic transitions (that is, phonon sidebands) usually dominate the emissions of Mn 4+ . In Fig. 4b , besides the weak ZPLs, we can observe several intense emission lines ranging from 630 to 637 nm, which originate from the electric dipole vibronic transitions induced by lattice vibrations with odd-parity. Consistently, at 3 K, phonon sidebands arising from the upper sublevel of 2 E g nearly disappeared (indicated by the vertical dashed lines in Fig. 4b ), and four sharp peaks centred at 630.81, 631.98, 634.68 and 635.98 nm were well resolved, respectively. Meanwhile, a much broader vibronic emission band was observed at ~647 nm. According to the group theory, there are six fundamental internal vibronic modes ν 1 (A 1g ), ν 2 (E g ), ν 3 (T 1u ), ν 4 (T 1u ), ν 5 (T 2g ) and ν 6 (T 2u ) of octahedral group with symmetry of O h . When the site symmetry of Mn 4+ is reduced from O h to D 3d , the triply degenerate modes ν 3 , ν 4 , ν 5 and ν 6 will further split into a doubly degenerate mode and a non-degenerate mode [48] . The vibronic modes coupled to the ZPLs of 2 E g → 4 A 2 are antisymmetric ν 3 (T 1u ), ν 4 (T 1u ) and ν 6 (T 2u ) [49] . Specifically, the two peaks at 630.81 and 631.98 nm are assigned to the 2 E g → 4 A 2 +ν 6 transitions, while the two peaks at 634.68 and 635.98 nm are attributed to the 2 E g → 4 A 2 +ν 4 transitions. The band at ~647 nm is due to the 2 E g → 4 A 2 +ν 3 transition, and two relatively sharp peaks centred at 646.10 and 646.85 nm can be identified. Besides, abundant weak peaks in the range of 0–400 cm −1 shifting from the R 1 line were observed ( Fig. 4c ). These emissions mainly arise from the external lattice vibronic modes coupled to the ZPLs. All vibronic frequencies identified from the 3-K emission spectra of K 2 TiF 6 :Mn 4+ were found consistent with those derived from their Raman and infrared spectra ( Supplementary Table 1 ) [34] , [48] . These results present additional evidence for the occupation of Mn 4+ ions in the sublattice of Ti 4+ . Unlike the 2 E g → 4 A 2 transition, the excited transitions of 4 A 2 → 4 T 1 , 4 T 2 are spin-allowed, which exhibit broadband feature at RT as a result of the overlapping of multi-order phonon sidebands induced by strong electron–phonon interaction. To probe the fine structure of these bands, we measured the excitation spectra of the K 2 TiF 6 :Mn 4+ (0.72 at.%) sample at 10 K ( Fig. 4d ). Particularly, the excitation band at ~468 nm was observed to split into several sharp peaks separated by spacing of ~550 cm −1 . These peaks belong to the totally symmetric ν 1 (A 1g ) vibronic progressions. The energy spacing of ~550 cm −1 is somewhat smaller than the energy of ν 1 (~618 cm −1 ). This discrepancy can be well explained by the fact that the vibronic frequencies derived from the excited state differ from those derived from the ground state, as the geometrical configurations are different in such two cases [49] . The energy levels of 3d 3 ions depend on the parameter D q , B and C , where D q is a parameter that characterizes the strength of the octahedral crystal field, while B and C are Racah parameters. We determined the values of these parameters from observed peak energies of 4 T 2 , 4 T 1 and 2 E g states in K 2 TiF 6 :Mn 4+ , 2121, 605 and 4061, cm −1 for D q , B , and C , respectively. Based on these parameters, we calculated the energies of other states 2 T 1 , 2 A 1 and 4 T 1 , located at 17,214, 36,316 and 28,698 cm −1 , respectively ( Supplementary Discussion ) [46] , [47] . On the other hand, the energy level of 2 T 1 can be experimentally determined by comparing the vibronic excitations of 4 A 2 → 2 T 1 , 2 E g at ~600 nm with the vibronic emissions of 2 E g → 4 A 2 at 10 K ( Fig. 4d,e ), that is, 17,107 cm −1 , which is consistent with the calculated energy (17,214 cm −1 ) of 2 T 1 . Note that the energy level of 2 T 1 had never been determined before this work. Abnormal temperature-dependent PL intensity It is well established that the PL intensity of most luminescent materials such as rare-earth-doped inorganic phosphors usually decreases with the rise of temperature due to the larger non-radiative transition probability at higher temperature. However, we observed an anomalous temperature-dependent PL behaviour in K 2 TiF 6 :Mn 4+ phosphors ( Supplementary Fig. 9 ). Typically, for the K 2 TiF 6 :Mn 4+ (0.72 at.%) sample, the total PL intensity due to the 2 E g → 4 A 2 transition at 300 K was found to increase about 40% relative to that at 10 K ( Fig. 5a ). For comparison, PL decays from 2 E g by monitoring the 631-nm emission at 10–300 K were measured ( Supplementary Fig. 10 ). The PL lifetime of 2 E g by single exponential fit was found to decrease from 11.9 ms at 10 K to 5.9 ms at 300 K ( Fig. 5b ). 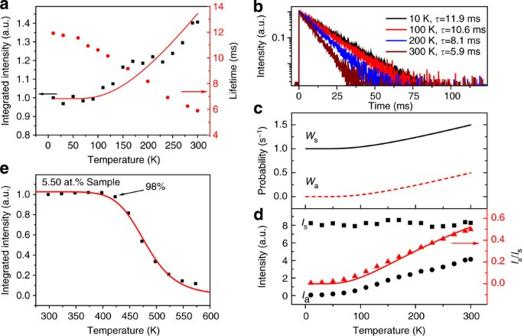Figure 5: Temperature-dependent photoluminescence (PL) intensity and dynamics in K2TiF6:Mn4+phosphor. (a) Integrated red PL intensity due to the2Eg→4A2transition and PL lifetime of the2Egstate as a function of temperature (10–300 K) for the K2TiF6:Mn4+(0.72 at.%) sample. The solid line represents the fitted result using the relationWab∝coth(ħω/2κT). (b) PL decays from the2Egstate at 10–300 K for the K2TiF6:Mn4+(0.72 at.%) sample. (c) Simulated temperature-dependent Stokes (Ws) and anti-Stokes (Wa) transition probabilities of2Eg→4A2by equations (1) and (2), respectively. (d) Measured PL intensities of ν6-mode-coupled Stokes (Is) and anti-Stokes (Ia) transitions of2Eg→4A2and the ratio ofIatoIsas a function of temperature at 10–300 K. The solid line represents the fitting result with the expression ofWa(T)/Ws(T). (e) Integrated red PL intensity due to the2Eg→4A2transition as a function of temperature (298–573 K) for the K2TiF6:Mn4+(5.50 at.%) sample. The solid line represents the fitting result with the expression ofIT/I0=[1+G·exp(−Ea/κT)]−1. a.u., arbitrary unit. Figure 5: Temperature-dependent photoluminescence (PL) intensity and dynamics in K 2 TiF 6 :Mn 4+ phosphor. ( a ) Integrated red PL intensity due to the 2 E g → 4 A 2 transition and PL lifetime of the 2 E g state as a function of temperature (10–300 K) for the K 2 TiF 6 :Mn 4+ (0.72 at.%) sample. The solid line represents the fitted result using the relation W ab ∝ coth( ħω /2 κT ). ( b ) PL decays from the 2 E g state at 10–300 K for the K 2 TiF 6 :Mn 4+ (0.72 at.%) sample. ( c ) Simulated temperature-dependent Stokes ( W s ) and anti-Stokes ( W a ) transition probabilities of 2 E g → 4 A 2 by equations (1) and (2), respectively. ( d ) Measured PL intensities of ν 6 -mode-coupled Stokes ( I s ) and anti-Stokes ( I a ) transitions of 2 E g → 4 A 2 and the ratio of I a to I s as a function of temperature at 10–300 K. The solid line represents the fitting result with the expression of W a ( T )/ W s ( T ). ( e ) Integrated red PL intensity due to the 2 E g → 4 A 2 transition as a function of temperature (298–573 K) for the K 2 TiF 6 :Mn 4+ (5.50 at.%) sample. The solid line represents the fitting result with the expression of I T / I 0 =[1+ G ·exp(− E a / κT )] −1 . a.u., arbitrary unit. Full size image To reveal the mechanism for this abnormal phenomenon, we conducted a thorough analysis of the temperature-dependent behaviour of the vibronic emissions, which contribute dominantly to the PL intensity of Mn 4+ . The temperature-dependent Stokes ( W s ( T )) and anti-Stokes ( W a ( T )) radiative transition probabilities of vibronic emissions can be expressed as [46] : where D is the proportional coefficient, ħω is the energy of the coupled vibronic mode, and κ is the Boltzmann constant. To demonstrate the effect of temperature on W s ( T ) and W a ( T ), we chose the most intense ν 6 -mode-coupled vibronic emissions. Figure 5c shows the simulated results of equations (1) and (2) in the temperature range of 0–300 K by setting ħω =230 cm −1 (the average energy of ν 6 mode) and D =1. Obviously, both Stokes and anti-Stokes transition probabilities increased with the rise of temperature. Correspondingly, the measured anti-Stokes emission intensity I a increased rapidly with temperature, whereas the Stokes emission intensity I s remained essentially unchanged ( Fig. 5d ). This can be attributed to the fact that the value of W a ( T ) increased more rapidly than that of W s ( T ) with the rise of temperature. To prove this, we fitted the data of I a / I s with the expression of W a ( T )/ W s ( T ) and observed a good agreement between experimental and fitted results ( Fig. 5d ). The PL lifetime of 2 E g is inversely proportional to the sum of radiative transition probability W r ( T ) (namely W s ( T )+ W a ( T )) and non-radiative transition probability W n ( T ). For the K 2 TiF 6 :Mn 4+ (0.72 at.%) sample, W n ( T ) is negligible at 10–300 K because the measured PL QY is 96% at 300 K. Therefore, the decrease of the PL lifetime with the increase of temperature should be owing to the enhanced W r ( T ) at elevated temperature ( Fig. 5a ). It should be noted that this mechanism is completely different from that in other luminescent materials, which are usually caused by increasing non-radiative transition probability with the rise of temperature. The PL intensity is proportional to the product of absorbed photons and PL quantum efficiency. Thus the effect of temperature on these two factors determines the temperature-dependent PL intensity. The quantum efficiency η of 2 E g can be expressed as W r ( T )/( W r ( T )+ W n ( T )). As W n ( T ) is negligible for the K 2 TiF 6 :Mn 4+ (0.72 at.%) sample at 10–300 K, the value of η can be approximated as a constant close to unit and it has no influence on the PL intensity with the change of temperature at 10–300 K. On the other hand, the transition probability W ab of the vibronic absorption of 4 A 2 → 4 T 2 is also temperature-dependent and proportional to coth( ħω /2 κT ) [46] . When taking these into account, the fitted PL intensity as a function of temperature agrees well with the observation ( Fig. 5a ). Hence, we infer that the main contribution to the incremental PL intensity at elevated temperature is ascribed to the increased absorption of excitation light by the sample. As expected, such an abnormal PL intensity behaviour should be concentration-independent. To prove this, we further measured the temperature-dependent PL intensities at 10–300 K for the 6.50 at.% sample, which displays a similar increase (~40%) in the PL intensity ( Supplementary Fig. 11 ). The working temperature of phosphors in LEDs could be much higher above RT. Usually, the remained PL intensity at 150 °C with respect to that at RT is used to evaluate the thermal stability of phosphors. The PL intensity of the K 2 TiF 6 :Mn 4+ (5.50 at.%) sample at 125 °C even increased about 2% when compared to that at 25 °C, as a result of the enhanced absorption as observed at 10–300 K. At 150 °C, the relative PL intensity of the sample remains 98% of that at 25 °C ( Fig. 5e ), showing clearly a better thermal stability than that of YAG:Ce 3+ phosphor [50] . However, above 175 °C, the emission intensity decreased rapidly due to the markedly increased non-radiative transition probability with further increase of temperature. We fitted the curve with the expression of I T / I 0 =[1+ G ·exp(− E a / κT )] −1 , where I 0 (intensity at T =0), G and activation energy E a are refined variables [51] . The K 2 TiF 6 :Mn 4+ (5.50 at.%) phosphor has an activation energy ( E a ) of ~0.70 eV, which is 3 times as high as that of nitride compounds (~0.25 eV) [52] . This verifies the excellent thermal stability of K 2 TiF 6 :Mn 4+ phosphors. Fabrication and performance of warm white LEDs To evaluate the device performance for the synthesized K 2 TiF 6 :Mn 4+ phosphor, we fabricated white LEDs with various CCTs by combining blue chips (455 nm), YAG:Ce 3+ yellow (YAG04, Intematix) or aluminate green phosphors (GAL535, Intematix), and the K 2 TiF 6 :Mn 4+ (5.50 at.%) red phosphor. The chromaticity coordinates of three typical LEDs with CCTs of 2,783, 3,556 and 5,954 K under a drive current of 60 mA, (0.4569, 0.4158), (0.3997, 0.3821) and (0.3224, 0.3416), are marked in CIE 1931 colour spaces, respectively, and all three colour points are laid on or close to the black body locus ( Fig. 6a ). Photographs of the as-fabricated LEDs and three lighted ones are shown in Fig. 6b–e . In accordance with the decrease of CCT, a pronounced warmer tone of the emitting light was observed, owing to the incremental red light component in the emission spectrum of LED. Electroluminescent spectra of the three LEDs reconfirm the sharp emission lines of Mn 4+ in K 2 TiF 6 phosphor and more red emitting component with the lower CCT ( Fig. 6f ). Table 2 compares the important photoelectric parameters such as CCT, CRI and luminous efficacy for the three LEDs. It is well known that a commercial white LED using a single YAG:Ce 3+ phosphor generally has a low CRI and high CCT, typically, R a <70 and CCT>5,000 K (ref. 53 ), which is unsuitable for indoor lighting. By adding K 2 TiF 6 :Mn 4+ red phosphor into the devices, warm white LEDs with R a >80 and CCT<4,000 K can be readily used for indoor lighting (LEDs 1 and 2, Table 2 ). Specifically, all the R9 values are positive, which suggest good rendition of the strong red colour. The luminous efficacies of these two LEDs are 110 and 116 lm W −1 under 60-mA drive current, respectively, which are much higher than that of the counterparts using nitride red phosphors (68 lm W −1 under 50-mA drive current) previously reported [54] . To the best of our knowledge, the luminous efficacy of LED 2 (116 lm W −1 , CCT=3,556 K) is the highest among warm white LEDs achieved on commercial blue chips in the literature. For LED 3, cool white light (CCT=5,954 K) with an ultrahigh CRI of R a =95 can be generated, where the phosphor blend is composed of aluminate green and K 2 TiF 6 :Mn 4+ red phosphors. To evaluate the current-dependent LED performance, we measured the luminous efficacies of the three LEDs under various drive currents of 20, 40, 60 (the rated current of blue chip), 80, 100 and 120 mA, respectively. The luminous efficacy of LED 1 was found to increase gradually from 110 to 124 lm W −1 when the drive current decreased from 60 to 20 mA ( Table 2 ). This is owing to the larger external quantum efficiency of the blue chip under lower drive current density [55] . Likewise, the luminous efficacies of LED 2 and 3 under 20 mA drive current reached as high as 132 and 135 lm W −1 , respectively. 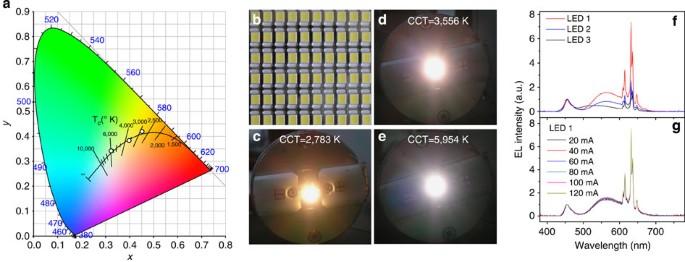Figure 6: Device performance of fabricated white LEDs based on K2TiF6:Mn4+red phosphor. (a) The chromaticity coordinates of three typical LEDs with correlated colour temperatures (CCTs) of 2,783, 3,556 and 5,954 K under a drive current of 60 mA in Commission Internationale de l'Éclairage (CIE) 1931 colour spaces. Photographs of the (b) as-fabricated LEDs and lighted ones with CCTs of (c) 2,783, (d) 3,556 and (e) 5,954 K, respectively. Electroluminescent (EL) spectra of (f) the three LEDs under 60-mA drive current and (g) LED 1 under various drive currents. All the spectra were normalized at the peak intensity at 455 nm. a.u., arbitrary unit. Figure 6: Device performance of fabricated white LEDs based on K 2 TiF 6 :Mn 4+ red phosphor. ( a ) The chromaticity coordinates of three typical LEDs with correlated colour temperatures (CCTs) of 2,783, 3,556 and 5,954 K under a drive current of 60 mA in Commission Internationale de l'Éclairage (CIE) 1931 colour spaces. Photographs of the ( b ) as-fabricated LEDs and lighted ones with CCTs of ( c ) 2,783, ( d ) 3,556 and ( e ) 5,954 K, respectively. Electroluminescent (EL) spectra of ( f ) the three LEDs under 60-mA drive current and ( g ) LED 1 under various drive currents. All the spectra were normalized at the peak intensity at 455 nm. a.u., arbitrary unit. Full size image Table 2 Important photoelectric parameters for three typical LEDs with different correlated colour temperatures (CCTs). Full size table Small colour fluctuation under varied excitation powers is crucial for the long-term service of LEDs. We found that the electroluminescent spectra of LED 1 under different drive currents remained essentially the same ( Fig. 6g ), indicative of very small colour fluctuation. The slight variation of the chromaticity coordinate, merely 0.0054 for CIE- x and 0.0048 for CIE- y , respectively, reconfirms the negligible colour fluctuation in LED 1. Theoretically, the PL intensity saturation might occur more likely in K 2 TiF 6 :Mn 4+ phosphor than in Ce 3+ - and Eu 2+ -activated phosphors due to the much longer PL lifetime of Mn 4+ (5.70 ms) than that of Ce 3+ and Eu 2+ (approximately tens of nanoseconds). Fortunately, as demonstrated in Fig. 6g , no PL intensity saturation was observed until the drive current reached 120 mA in LED 1, which indicates the potential use of our phosphors in high power LEDs. In summary, we have developed a novel cation exchange strategy for the synthesis of micrometre-sized K 2 TiF 6 :Mn 4+ phosphor with an unusually fast rate, where 67% of the Mn 4+ ions in the precursor solution were found to substitute for the Ti 4+ ions within 3 min. The synthesized K 2 TiF 6 :Mn 4+ red phosphor shows an extremely high PL QY up to 98%, which is superior to those of rare-earth (oxy)nitride red phosphors such as Ca-α-SiAlON:Eu 2+ (QY=70.5%) and CaAlSiN 3 :Ce 3+ (QY=80%) [18] , [19] . The proposed approach shows the advantages of higher production yield, much less HF solution consumption and shorter preparation time than those previously reported, thus paving the way for mass production of this phosphor. Furthermore, we have demonstrated the universality of this approach through the successful syntheses of other Mn 4+ -activated fluoride phosphors such as K 2 SiF 6 :Mn 4+ , NaGdF 4 :Mn 4+ and NaYF 4 :Mn 4+ . More importantly, the K 2 TiF 6 :Mn 4+ phosphor exhibited the most intense excitation band at ~468 nm with a bandwidth of ~50 nm, which is perfect for blue-chip excitation. The spectral overlap between this excitation band and the emission band of YAG:Ce 3+ is negligible, hence the problem of re-absorption that occurred in LEDs based on (oxy)nitride red phosphors can be avoided. Furthermore, the phosphor exhibited sharp red emissions at ~630 nm, thereby rendering a higher LER in warm white LEDs as compared to (oxy)nitride red phosphors that show substantial emission spreading into deep red spectral region. By means of low-temperature high-resolution spectroscopy, the detailed electronic/vibronic structure of Mn 4+ ions in K 2 TiF 6 host has been elaborated. The observed energy level splittings of Mn 4+ , with a crystallographic site symmetry of D 3d , were found in good agreement with that calculated theoretically, which provides additional evidence for the residence of Mn 4+ in the sublattice of Ti 4+ through cation exchange. Based on PL dynamics, PL QY and theoretical analysis, we have revealed the mechanism for abnormal dependence of PL intensity on the temperature in K 2 TiF 6 :Mn 4+ (an increase of ~40% in the PL intensity at 300 K relative to that at 10 K). It has been corroborated that the increased absorption of excitation light by the sample contributed dominantly to the incremental PL intensity with the rise of temperature. Finally, by integrating this phosphor with commercial YAG:Ce 3+ yellow phosphor and 455-nm blue chip, we have fabricated a warm white LED with high CRI ( R a =81), low CCT (3,556 K) and a record-high luminous efficiency of 116 lm W −1 under rated 60-mA drive current. The LEDs also show excellent chromaticity coordinate stability with the drive current varied from 20 to 120 mA. These findings show great promise of K 2 TiF 6 :Mn 4+ as commercial red phosphor in warm white LEDs, and open up new avenues for the exploration of novel non-rare-earth red emitting phosphors. Chemicals and materials K 2 TiF 6 (≥99.95 %), K 2 SiF 6 (≥99.999 %) and HF solution (49 wt.%, ≥99.99998 % metals basis) were purchased from Aladdin Chemistry, China. The K 2 MnF 6 crystals were prepared based on Bode’s method [56] . All the chemicals were used directly without further purification. Synthesis of K 2 TiF 6 :Mn 4+ phosphor A cation exchange approach was employed for the synthesis of K 2 TiF 6 :Mn 4+ microcrystals. To demonstrate this, we described the preparation procedure for the K 2 TiF 6 :Mn 4+ (0.72 at.%) sample. Typically, 0.0360, g of K 2 MnF 6 powders were first dissolved in 1.8 ml of HF solution (49 wt.%). Then, the obtained solution was mixed with 4.9640, g of K 2 TiF 6 powders under stirring for 20 min to form a uniform muddy mixture, which was subjected to drying at 70 °C for 3 h in an oven. The final product showed a uniform yellow tint under natural light illumination. Other four samples with Mn 4+ concentrations of 1.40, 2.10, 5.50 and 6.50 at.% were prepared following the same procedure. A proof-of-concept experiment was designed to reveal the occurrence of cation exchange in the above approach. First, 0.0452, g of K 2 MnF 6 powders were dissolved in excess of HF solution (49 wt.%, 0.8 ml), which afforded a clear brown solution. Then, 0.7548, g of K 2 TiF 6 powders were added to the solution (the atom percent of Mn is 5.50 %). The quantity of the added K 2 TiF 6 powders was small to maintain good fluidity of the solution, thus facilitating the separation of the products by vacuum filtration. Finally, after cation exchange for 3 min under stirring, the undissolved powders in the solution (0.5796, g) were isolated instantly through vacuum filtration, followed by drying at 70 °C for 3 h. The colour of the mixture solution was observed to change from brown to light-yellow. Accordingly, the colour of the powders changed from white to yellow after cation exchange. Structural and optical characterization Powder XRD patterns of the K 2 TiF 6 :Mn 4+ samples were measured by an X-ray diffractometer (DMAX 2500PC, Rigaku) at an interval of 0.02° with the speed of 2° min −1 with Cu Kα1 radiation ( λ =0.154187, nm). The unit cell refinements were accomplished by the JADE software. The morphologies of the samples were characterized by a scanning electron microscope (JSM-6700F). Scanning transmission electron microscopy and energy dispersive spectroscopy analyses were performed on a TECNAI G 2 F20 TEM operated at 200 kV. Compositional analyses were performed using an ICP–AES (Ultima2). The RT excitation and emission spectra and PL decays were measured with an Edinburgh Instrument FLS920 spectrometer equipped with both continuous (450 W) and microsecond pulsed xenon (Xe) lamps. For temperature-dependent experiments at 10–300 K, the samples were mounted on an optical cryostat (10–350 K, DE202, Advanced Research Systems). The high-resolution spectral measurements at 3–30 K were carried out using a monochromator with 1-m focal length (1,000 M, Jobin-Yvon) equipped with a photomultiplier tube (R943-02, Hamamatsu), and the samples were mounted on an optical cryostat (3–300 K, SHI-950, Janis Research). To investigate the PL thermal stability at 298–573 K, the samples were placed on a thermal stage (77–873 K, THMS 600, Linkam Scientific Instruments) and a fibre coupled spectrometer (QE 65000, Ocean Optics) was used to record the emission spectra of the sample excited by a 455-nm diode chip. For PL QY measurement, the samples were put inside an optical integrating sphere coupled to the FLS 920 spectrometer. A standard tungsten halogen lamp was used to correct the optical response of the instrument. LEDs fabrication and performance measurement White LEDs with various CCTs were fabricated by combining blue chips (455 nm, 180 mW, 60 mA, Tekcore), YAG:Ce 3+ yellow (YAG04, Intematix) or aluminate green phosphors (GAL535, Intematix) and the K 2 TiF 6 :Mn 4+ (5.50 at. %) red phosphor. The blue chip was first fixed on the bottom of a reflector. The phosphors were mixed with silicone thoroughly and the obtained phosphor–silicone mixture was coated on the surface of the LED chips to produce white LEDs. The photoelectric properties of the fabricated devices were measured by an integrating sphere spectroradiometer system (LHS-1000, Everfine). The LEDs were operated at 3.0 V with various drive currents of 20, 40, 60, 80, 100 and 120 mA, respectively. The spectral power distributions of the LEDs were measured by a corrected spectrometer to calculate their values of CCT and CRI (ref. 57 ). The luminous efficacy was measured as the ratio of luminous flux (lm) output to the input electrical power (W) of the LEDs. The CCTs of three typical fabricated LEDs were 2,783 (LED 1), 3,556 (LED 2) and 5,954 K (LED 3) under a drive current of 60 mA, respectively. For LEDs 1 and 2, the phosphor blend was composed of YAG04 yellow and K 2 TiF 6 :Mn 4+ (5.50 at. %) red phosphors. For LED 3, the phosphor blend was composed of GAL535 green and K 2 TiF 6 :Mn 4+ (5.50 at.%) red phosphors. The mass percentages of red phosphor in the phosphor blends were 70, 61 and 50% for LEDs 1–3, respectively. How to cite this article: Zhu, H. et al. Highly efficient non-rare-earth red emitting phosphor for warm white light-emitting diodes. Nat. Commun. 5:4312 doi: 10.1038/ncomms5312 (2014).